Quantification of nanowire penetration into living cells High-aspect ratio nanostructures such as nanowires and nanotubes are a powerful new tool for accessing the cell interior for delivery and sensing. Controlling and optimizing cellular access is a critical challenge for this new technology, yet even the most basic aspect of this process, whether these structures directly penetrate the cell membrane, is still unknown. Here we report the first quantification of hollow nanowires—nanostraws—that directly penetrate the membrane by observing dynamic ion delivery from each 100-nm diameter nanostraw. We discover that penetration is a rare event: 7.1±2.7% of the nanostraws penetrate the cell to provide cytosolic access for an extended period for an average of 10.7±5.8 penetrations per cell. Using time-resolved delivery, the kinetics of the first penetration event are shown to be adhesion dependent and coincident with recruitment of focal adhesion-associated proteins. These measurements provide a quantitative basis for understanding nanowire–cell interactions, and a means for rapidly assessing membrane penetration. High-aspect ratio nanostructure platforms are rapidly developing as tools to couple inorganic materials to cells and access the cell interior. Since 2004, vertical nanowire arrays and similar structures have been explored as systems to deliver a variety of cargoes to various cell types [1] , [2] , [3] , act as optical point sources [4] and measure cellular electrical activity [5] . These systems are particularly promising as delivery systems for perturbing cellular behaviour, as direct intracellular delivery of cargo avoids endosomal entrapment and degradation [6] , [7] and is largely agnostic to the identity of the material being delivered [8] and possibly even the cell type receiving the material [9] . Despite the growing importance of this method, the fundamental mechanisms are still unclear, including whether the nanowires actually penetrate the cell membrane. Enhanced endocytosis and tight membrane engulfment may produce similar results, and several structural characterization studies [10] , [11] , [12] have found no evidence of membrane rupture and intracellular access near nanowires. Electrophysiological measurements with nanowires have also shown that trans-membrane access requires external inducement such as electroporation [5] , [13] , [14] . On the other hand, other groups have reported efficient delivery of RNA, DNA and proteins into a variety of cell types [8] , [15] , [16] , [17] by simply plating cells onto nanowires. Recently, nanowires have been used to assay intracellular content [18] , thus demonstrating intracellular access albeit by physically pressing cells using a ‘sandwich’ method. These conflicting results lead to significant questions about how nanowires interact with the cell membrane, whether the membrane is penetrated, the number of nanowires that actually penetrate or become engulfed and the role of nanowire surface characteristics in penetration. Forward progress of nanowire–cell interface technology is limited until these questions can be answered, but the extent to which nanowires penetrate the cell is still difficult to characterize by existing methods. When solid nanowires are used for reagent delivery to determine whether the cell has been penetrated, endocytosis creates background uptake and complicates analysis [8] , [16] . With these techniques, delivery acts as a proxy for penetration and cannot reveal where penetration took place, or the percentage of nanowires that achieved intracellular access. Confocal microscopy of the cell membrane can image the interface in real time, but has limited resolution and may miss small ruptures in the membrane that allow material transfer [8] , [12] . Electron microscopy techniques have sufficient resolution, but require extensive sample processing before imaging and have relatively small sample sizes so that infrequent rupture events could be missed [10] . The inability to effectively observe when and where molecules are delivered obfuscates the underlying processes, making it difficult to distinguish nanowire penetration delivery from other possible delivery mechanisms. Here we use a new platform to quantitatively determine the percentage, spatial location and kinetics of high-aspect ratio hollow nanowires—nanostraws—that actually penetrate through the cell membrane. As shown in Fig. 1a , nanostraws are grown en masse on a track-etched membrane and are similar in geometry to typical vapour–liquid–solid nanowire arrays [16] . Unlike solid nanowires, each 100-nm diameter nanostraw spans the thickness of the supporting membrane, allowing molecules to pass from one side of the membrane to the other through the nanostraw. This provides dynamic control of chemical delivery simply by regulating the solution composition. If the nanostraw penetrates the cell, molecules can diffuse through the nanostraws and into the cytoplasm ( Fig. 1b ). The diffusive nature of molecular delivery into the cytosol precludes endocytosis uptake or engulfment, and the accumulation of diffused molecules allows even small ruptures in the cell membrane to be sensed using optical microscopy, eliminating the ambiguity owing to limited imaging resolution or small sampling size. The nanostraws that penetrated green fluorescent protein (GFP)-expressing cells were visualized by observing delivery of a fluorescence-quenching ion at prescribed time points. Penetrant nanostraws led to distinct quenching ‘spots’ that were quantified to determine the number of fluidic cytosolic interfaces formed for each cell ( Fig. 1c ). We discovered that of the hundreds of nanostraws in contact with each cell, approximately one in fifteen nanostraws (7.1%) is able to penetrate an adherent cell, and these nanostraws retain cytosolic access over time for diffusive delivery of multiple species in sequence. These results help resolve the discrepancy between microscopy studies concluding that nanowires are unable to penetrate cells [10] , [12] and experimentally observed material delivery [8] , [16] , as penetration is an infrequent, but regularly occurring, event. The time-resolved delivery of the nanostraw technique also permits more complex patterns of molecular delivery to enable study of the early stages of penetration, which shows that the time scale of penetration ranges from hours for unmodified surfaces to 5 min for an adhesion-promoting surface. Finally, we observe adhesion proteins localizing to nanostraws, indicating a possible mechanism for penetration. These experiments are the first in situ delivery observations of what is fast becoming a powerful enabling technology [13] , [15] , [19] , [20] , [21] , [22] , [23] , [24] and the results can be used to tailor nanowire systems to enhance electrical recordings, streamline cellular delivery and standardize cell penetration. 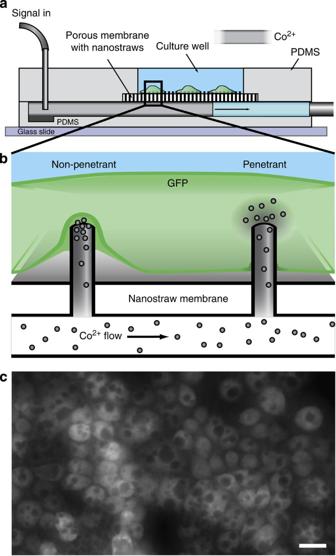Figure 1: An ionic delivery assay designed to probe nanostraw cell penetration. Nanostraw membranes are integrated into a microfluidic device (a) For each cell plated in the device, there are many nanostraw interfaces that may either be non-penetrant or penetrant (b). When the nanostraws penetrate into the cell membrane, the Co2+ions in the solution below are able to directly enter the cell via passive diffusion and quench GFP fluorescence (c, scale bar, 20 μm). Figure 1: An ionic delivery assay designed to probe nanostraw cell penetration. Nanostraw membranes are integrated into a microfluidic device ( a ) For each cell plated in the device, there are many nanostraw interfaces that may either be non-penetrant or penetrant ( b ). When the nanostraws penetrate into the cell membrane, the Co 2+ ions in the solution below are able to directly enter the cell via passive diffusion and quench GFP fluorescence ( c , scale bar, 20 μm). Full size image In situ observation of cell penetration We developed a simple assay for visualizing nanostraw penetration through the membrane. Chinese hamster ovary (CHO) cells constitutively expressing enhanced GFP (eGFP) were plated for 24 h on polyornithine-coated nanostraw membranes in 5-mm diameter circular wells (10k cells per well) with a 0.5-mm-wide delivery channel running below the membrane ( Fig. 1a ). The distribution of eGFP throughout the cell was relatively uniform based on the fluorescence intensity, with higher brightness in the soma due to its greater height. We then added a 200 mM Co 2+ solution to the delivery channel, allowing Co 2+ ions to enter cells via nanostraws measured to be ~100 nm in diameter and ~1 mm in height. This high concentration in the subphase was necessary owing to the limited transport through the narrow nanostraws. GFP fluorescence is locally quenched [25] around the penetrating nanostraw as Co 2+ accumulates within the cell, producing a quenching pattern of dark spots ( Fig. 1c ). Intracellular access (that is, a penetrating nanostraw) is necessary to induce the observed quenching pattern ( Fig. 1b ), as control experiments with externally delivered Co 2+ at the same concentration do not quench cell fluorescence. In addition, the presence of Co 2+ near the cell through a nanostraw is insufficient for quenching, since we observe that the majority of nanostraws under the cell do not produce quenching spots. Moreover, quenching spots grow in size over time in a Guassian profile, consistent with Co 2+ diffusing within the cell and quenching the local cytosolic pool of fluorescent molecules ( Supplementary Discussion ). Therefore, each microscale ‘spot’ corresponds to a nanostraw penetration and cytosolic delivery event. As long as Co 2+ solution is present in the fluidic channel beneath the membrane, Co 2+ ions can diffuse through the nanostraws and accumulate inside cells. As shown in Fig. 1c , the dark spots eventually grow to a size easily observed by epifluorescence optical microscopy, allowing us to record the subwavelength penetration event with standard tools. Live cell imaging of delivery and quenching was performed with a × 20 objective, revealing a multitude of dark, roughly circular quenching spots. Quenching already fluorescent cells avoided the background intensity, endocytotic uptake challenges and frequent washing steps of previous fluorescent dye uptake experiments [16] . The current assay circumvents these primary drawbacks of dye or indicator delivery, and provides both temporal and spatial mapping of penetrating nanostraw locations in situ . Control experiments of Co 2+ delivery to cells on nanoporous membranes without nanostraws or on conventional polystyrene culture dishes did not show quenching owing to the low membrane permeability of Co 2+ in the absence of ionophores [26] , [27] . Furthermore, in these experiments Co 2+ was restricted to a microfluidic channel underneath the nanostraw membrane, and cells that were situated off the channel (which did not receive Co 2+ but were still located on top of nanostraws) were unaffected during the delivery time ( Supplementary Movie 1 ). Replacing Co 2+ with an equivalent concentration of another divalent ion (Mg 2+ , Ca 2+ ) was also ineffective for fluorescence quenching, which confirms that osmotic effects such as localized membrane rupture are not significant. The overall cell exposure to Co 2+ should be kept to a minimum (<30 min) however, as Co 2+ is known to be cytotoxic [28] , [29] even without internalization; after ~60 min we observe cell death and cell-wide fluorescence loss. Quantification of nanowire–cell penetration and delivery The quenching of cytosolic fluorescence produces a pattern of spots in the cells, each one of which corresponds to a membrane penetration event ( Fig. 2a ). Essentially every cell (>95%) is penetrated by one or more nanostraws, with an average of 10.7±6 penetration events per cell ( n =252, s.d.) as shown in Fig. 2b . When compared with the number of nanostraws under each cell (31±5 nanostraws per 100 μm 2 , ~150 nanostraws per cell), the penetration rate was 7.1±2.7 percent, or 1 in 14–15 nanostraws. This percentage is fairly low, making these events difficult to detect using a small sampling size technique such as electron microscopy, or a lower density array of nanowires. On normalization to cell area to remove cell size variation, the average was 0.022±0.009 spots per μm 2 ( Fig. 2c ) with a more Gaussian distribution compared with the raw number of penetrations per cell. There was little correlation between cell area and the density of spots ( Fig. 2d , R 2 =0.1294), suggesting that each penetration event is stochastic and independent of its neighbours, and any co-operativity or avidity effects are weak. Quenching spots are difficult to resolve before they grow to a size over 1 μm (which is also the average spacing of nanostraws) so it is possible that some quenching spots, especially oblong or ellipsoidal spots, arise from two or more penetrating nanostraws in close proximity. Given that almost all spots are well separated with only a few overlapping, it is statistically unlikely that many of the observed spots are due to multiple penetrations at the submicrometer scale, although our resolution cannot rule out this possibility. 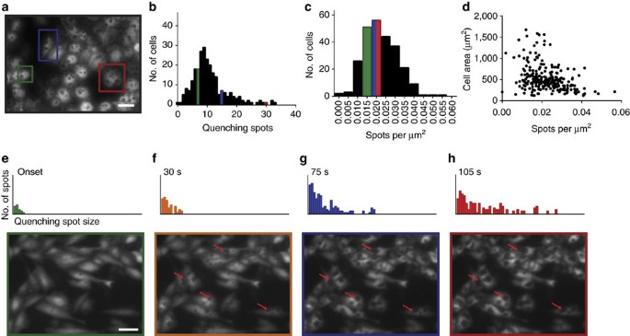Figure 2: Quenching spots indicate sites of nanostraw penetration. During Co2+delivery, quenching spots grow in size as Co2+accumulates above a penetrating nanostraw. Spots were counted (a,n=252, scale bar, 25 μm) to determine the number of spots per cell (b), the density of spots per cell (c) and the dependence of spot density on cell area (d). The largest cells generally had more spots (red) than intermediate sized cells (blue) and small cells (green), but the actual density of spots was largely independent of cell area (c,d). The number of spots and their size increased (e–h, scale bar, 40 μm) as spots accumulated enough Co2+to be observed. Figure 2: Quenching spots indicate sites of nanostraw penetration. During Co 2+ delivery, quenching spots grow in size as Co 2+ accumulates above a penetrating nanostraw. Spots were counted ( a , n =252, scale bar, 25 μm) to determine the number of spots per cell ( b ), the density of spots per cell ( c ) and the dependence of spot density on cell area ( d ). The largest cells generally had more spots (red) than intermediate sized cells (blue) and small cells (green), but the actual density of spots was largely independent of cell area ( c , d ). The number of spots and their size increased ( e – h , scale bar, 40 μm) as spots accumulated enough Co 2+ to be observed. Full size image As the number of nanostraws per unit area is relatively uniform over the 10–30-μm diameter of the cells, the minor variability owing to the random placement of the nanostraws was not expected to account for the differences in penetration observed. Nanostraw density variations alone can account for a s.d. of ±0.002 penetration events per μm 2 , yet we observed a s.d. of ±0.009 events per μm 2 , demonstrating that differences between cells, not the distribution of the nanowires, create the distribution in cell penetration. Among these differences may be factors such as individual cell motility and health, but cell surface area does not appear to be a key factor. While the penetration likelihood was generally uniform over the entire cell area, the amount of material delivered was not. The quantity of Co 2+ delivered was reflected in the rate of spot growth during delivery, which was substantially different between the soma and periphery. Quenching spot growth over 105 s was traced for spots that exceeded a minimum size threshold (15.7 mm 2 ) in Fig. 2e to 2 h. Many spots remained relatively small over the time period, but the average spot size steadily increased due to a small number of rapidly growing spots ( Supplementary Fig. 1 ). Generally, the amount of material delivered was largest at the cell soma, where the majority of the cell’s volume is located, and smallest at the cell periphery. This suggests that after membrane penetration, spot growth is limited by the accessible volume of cytosol above a penetrating nanostraw, which decreases closer to the cell periphery. For example, nanowires near the periphery may be in contact or close proximity to the upper membrane, limiting mass flux, while those within the soma are uninhibited and deliver more of the cargo. This has important implications for gene or protein delivery with nanostraws, which may be much less effective if confined to the cell periphery. Interestingly, some of the nanostraws appeared to penetrate the Hoechst-labeled nuclei directly ( Supplementary Fig. 2 ). In these cases the entire nucleus would quench rapidly at a subminute time scale, which was distinct from the slower spot growth observed in the cytosol. Nuclear quenching was quite rare, observed in <5% of cells, and was accompanied by a gradual loss of total cellular fluorescence. These observations suggest that of nanostraws that are able to penetrate into cells, a small minority have access to internal subcellular compartments such as the nucleus. Alternating delivery through nanostraw interfaces The fluidic exchange possible with nanostraws provides temporal control over delivery as compared with solid nanowires, which we use to demonstrate the stability of nanostraw cytosolic access. In this assay, molecular delivery is switched between Co 2+ and 100 mM ethylenediaminetetraacetic acid (EDTA), a small molecule chelator of divalent cations. When EDTA was delivered after Co 2+ quenching, we observed full or partial recovery of quenching spots to green fluorescence ( Fig. 3a ; Supplementary Discussion ; Supplementary Fig. 3 ). This process could be repeated over time ( Supplementary Movie 1 ), leading to cycles of quenching and recovery (additional cycling led to cell death due to overexposure to Co 2+ ). The observed quenching and restoration of fluorescence occurred quickly, on a minute time scale. Nanostraw cytosolic access was stable over this time period and, given that these cells had been cultured on the nanostraw membrane for 24 h preceding testing, probably much longer. Spots were observed to form at the same location from cycle-to-cycle ( Fig. 3b–g , red arrows) and spots combined with each other when grown to sufficient size (blue arrows). The recurring formation of spots at the same location strongly suggests that a single penetrating nanostraw provides long-term access to the cytosol at each instance, and the observation that spots grow and combine with other spots demonstrates that penetrating nanostraws access the same, shared compartment of cytosolic GFP. 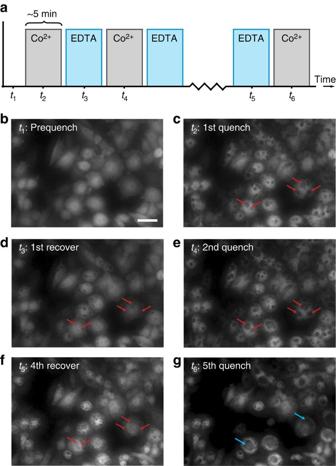Figure 3: Alternating intracellular reagent delivery. Solutions of Co2+or an ethylenediaminetetraacetic acid (EDTA) chelator were alternately pumped into the device for ~5 min (a) beginning with the prequenched state (b, scale bar, 25 μm). Quenching spots formed during the first quenched state (c), and were mostly recovered during the first recovery (d). During the second recovery (e), most quenching spots were directly associated with a spot from the first recovery (red arrows). After later recovery (f) and quench cycles (g), the recovery steps become insufficient to fully restore fluorescence. During later quench cycles, neighbouring spots grew large enough to combine with each other, demonstrating that a single pool of cytosolic GFP was quenched (blue arrows). Figure 3: Alternating intracellular reagent delivery. Solutions of Co 2+ or an ethylenediaminetetraacetic acid (EDTA) chelator were alternately pumped into the device for ~5 min ( a ) beginning with the prequenched state ( b , scale bar, 25 μm). Quenching spots formed during the first quenched state ( c ), and were mostly recovered during the first recovery ( d ). During the second recovery ( e ), most quenching spots were directly associated with a spot from the first recovery (red arrows). After later recovery ( f ) and quench cycles ( g ), the recovery steps become insufficient to fully restore fluorescence. During later quench cycles, neighbouring spots grew large enough to combine with each other, demonstrating that a single pool of cytosolic GFP was quenched (blue arrows). Full size image The diffusive nature of long-term nanostraw access and fluorescence quenching was confirmed by the shape and intensity of quenching spots during Co 2+ quenching and subsequent EDTA recovery. The line profiles and surface plots of the fluorescence intensity as a function of time are shown in Supplementary Fig. 4a–d . Consistent with a diffusive mechanism, Co 2+ delivery reduces local fluorescence intensity in a Gaussian profile. This is more easily observed when plotted as a reduction in fluorescence intensity, a direct proxy for Co 2+ concentration, as shown in Supplementary Fig. 4e–j , where the Gaussian shape is clearly apparent. After EDTA delivery, the majority of quenched GFP is restored to resemble the prequenched state. The fluorescence switching after repeated Co 2+ /EDTA cycles became less responsive, likely due to Co 2+ toxicity or eventual loss of fluidic access. When cells stopped responding to quenching after repeated cycles, they were often observed to lose their fluorescence suddenly. The sudden loss of fluorescence sometimes occurred separately in the cell cytosol and the nucleus ( Supplementary Fig. 5 ). The quantitative amount of Co 2+ necessary to induce quenching is unclear at this point, as the nature of the Co 2+ –GFP interaction is unknown and many of the ions may bind to other cytosolic components. The relative differences in size and expansion rate between spots can be attributed to local differences in Co 2+ delivery rate (for instance due to membrane or protein occlusion), or different distribution of cytosolic components. Kinetics of nanostraw penetration Since Co 2+ quenching provides a rapid in situ penetration assay, the appearance of the spots can also be used to study penetration kinetics. The time frame for nanostraw penetration was ascertained by adding free-floating cells into the solution above a polyornithine-coated nanostraw device ( Fig. 4a ) and observing in real time as they settled onto the nanostraws ( Fig. 4b ). The time at which each cell made contact with the nanostraws was recorded, and then a Co 2+ pulse (500 mM) was delivered at either 30 or 45 min ( Fig. 4c ). Successful penetration (as defined by formation of at least one quenching spot within a cell) was then compared with the cell adherence time before the Co 2+ pulse ( Fig. 4d ; Supplementary Fig. 6 ). This procedure avoided complications owing to the presence of Co 2+ that may have interfered with cell attachment. 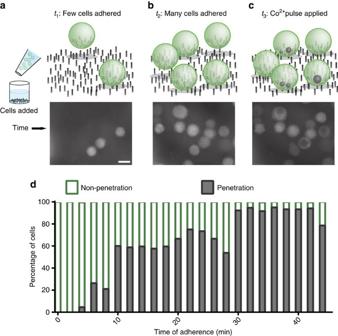Figure 4: Kinetics of penetration determined by ionic delivery. The Co2+penetration assay was applied to cells immediately as they were plated on nanostraws to determine penetration kinetics. First cells were added to a device (a, scale bar, 10 μm) and tracked as they contacted the nanostraws (b). Eventually a pulse of Co2+was added to the device, resulting in quenching spots forming within the cells (c). Over 30 min, cells became more likely to be penetrated at least once (d). Figure 4: Kinetics of penetration determined by ionic delivery. The Co 2+ penetration assay was applied to cells immediately as they were plated on nanostraws to determine penetration kinetics. First cells were added to a device ( a , scale bar, 10 μm) and tracked as they contacted the nanostraws ( b ). Eventually a pulse of Co 2+ was added to the device, resulting in quenching spots forming within the cells ( c ). Over 30 min, cells became more likely to be penetrated at least once ( d ). Full size image Three general regimes were observed for cell penetration. For cells with <10 min adherence, penetration was extremely unlikely (11% of cells). Cells adhering between 10 and 30 min experienced an intermediate regime of penetration (65%), while cell access was highly likely with 30 min or more of cell adhesion (92%). The likelihood of cell penetration roughly follows a sigmoidal curve, and the three regimes agree with previous estimates of time required for successful material delivery (~30 min) [8] . Some cells were observed to swell during Co 2+ delivery ( Supplementary Fig. 7 ), which is consistent with osmotic swelling as the cytosol becomes hypertonic relative to extracellular solution. We observe this phenomenon during this settling experiment but not in cells plated for 24 h, where cells are well adhered. The shape of the fluorescence quenching spots at early stages was almost always circular, in contrast to the sometimes polygonal shape of spots formed in well-adhered cells. The observation of circular spots reaffirms the diffusive hypothesis of direct intracellular delivery, as the expanding circles are representative of more spherically symmetric accumulations of Co 2+ . Role of cell adhesion in nanostraw penetration Nanostraw penetration depends strongly on the cell’s adherence time, suggesting that cellular adhesion to the nanostraw substrate is an important factor in the mechanism of penetration. The state of extracellular matrix elements and cell adhesion has already been implicated in cell membrane penetration by other techniques [30] , [31] . To modulate cell adhesion, nanostraw substrates were incubated in 10 μg ml −1 fibronectin, a well-characterized cell adhesion molecule [32] , in addition to the standard polyornithine coating. After culturing the cells for 24 h, Co 2+ was again introduced. The nanostraw penetration success rate increased to 12.1% ( n =165) compared with 7.1% without fibronectin, a 70% increase. In addition, the total number of spots per cell increased from 7.1±2.7 to 11.6±4.9, and spot density grew from 0.022±0.009 to 0.038±0.014 spots μm −2 , while the number of cells with at least one penetration spot was essentially 100%. Clearly, enhancing cell adhesion substantially increased the likelihood of penetration in a statistically significant manner ( P <0.005). In the absence of both adhesion promoters, polyornithine and fibronectin, the incidence of spots per cell and spot density were 6.3±3.1 and 0.018±0.007 μm −2 , respectively, for a nanostraw penetration success rate of 6.1% ( n =439). Nanostraws are still able to penetrate cells when unmodified, albeit less effectively. This observation is not surprising, as after 24 h most adherent cells are able to assemble and remodel extracellular matrix elements [33] . The effect of adhesion promotion is most easily observed in the kinetics of penetration. When the nanostraws were coated with fibronectin before plating and the kinetic quenching assay was performed, the time scale for nearly 100% cell penetration shifted markedly from 30 to 5 min ( Supplementary Fig. 8 ). Successful penetration was nearly universally observed for any cells that adhered for >5 min and well-spread cells were commonly observed. In the absence of fibronectin and polyornithine, nanostraw penetration at short time scales drops precipitously. Cell spreading was rare at times up to an hour, and penetration occurred in only ~20% of cells with an adherence time of 1 h or less. In contrast to the minor drop in penetration efficiency described earlier after 24 h of cell culture when substrates were uncoated, there is a drastic deceleration in penetration kinetics at short time scales. This shows that cell adhesion is critical for penetration, and that natural cell adhesion-driven penetration can be enhanced ectopically. Biomolecular adhesion correlates to penetration Cellular adhesion is an important driver of cell penetration, and we expected to see the effects of adhesion enhancement reflected in cellular structure including focal adhesion elements and cytoskeleton. To follow development of adhesion complexes concurrently with spot formation, eGFP-paxillin was transfected into CHO cells, which were then plated on nanostraws, fixed and stained with phalloidin conjugated to Alexa-Fluor 568. Paxillin is an important mediator of cell-substrate adhesion and phalloidin is used to label F-actin, an important cytoskeletal element [34] , [35] . When cells were plated on nanostraws, paxillin and F-actin organized into characteristic puncta ( Fig. 5a,b ), in contrast to typical features observed on flat membranes ( Fig. 5c,d ). 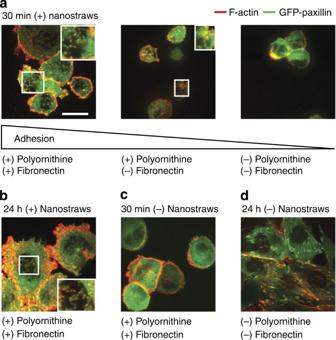Figure 5: Cell adhesion correlated with penetration. Biomolecular adhesion markers indicate that cells interact strongly with nanostraws. During initial cell contact after 30 min, enhanced cell adhesion was associated with cell spreading and actin and paxillin colocalization (a, scale bar, 10 μm). These features were lost as adhesion was decreased. The mature state after 24 h of adhesion showed stress fibre formation as well as actin and paxillin colocalization (b). Without nanostraws, some actin stress fibres appeared but no paxillin features were observed (c). The mature state without nanostraws featured paxillin puncta attached to stress fibres, but no colocalization (d). Figure 5: Cell adhesion correlated with penetration. Biomolecular adhesion markers indicate that cells interact strongly with nanostraws. During initial cell contact after 30 min, enhanced cell adhesion was associated with cell spreading and actin and paxillin colocalization ( a , scale bar, 10 μm). These features were lost as adhesion was decreased. The mature state after 24 h of adhesion showed stress fibre formation as well as actin and paxillin colocalization ( b ). Without nanostraws, some actin stress fibres appeared but no paxillin features were observed ( c ). The mature state without nanostraws featured paxillin puncta attached to stress fibres, but no colocalization ( d ). Full size image Applying cell adhesion coatings to nanostraws accelerated formation of these puncta, apparently in parallel to the enhancement of adhesion described previously. On fibronectin and polyornithine-coated nanostraws, cells were well spread after 30 min, some F-actin filaments could be observed and F-actin and paxillin puncta were observed at the cell-substrate height level, indicating recruitment of these proteins by nanostraws and frequent colocalization ( Fig. 5a ). With a less-adherent coating (polyornithine only) and the same adhesion time, the cell density was reduced and cell spreading and actin filaments were no longer observed, but the puncta could still be observed. Without coating, cells became very scarce and the basal side of the cell was poorly defined in the z -direction, indicating that the cell-substrate contact was still poor and the cell was primarily spherical. Finally, puncta were rare or ill-defined, in marked contrast with the doubly coated nanostraws. The cells eventually reached a mature adhesion state on nanostraws as observed in cells adhered for 24 h. At this advanced stage, many coincident paxillin and F-actin fluorescent puncta and F-actin stress fibres were readily observed ( Fig. 5b ). In marked contrast, when cells were plated on flat membranes without nanostraws, the coincident paxillin/F-actin puncta did not appear at short time spans ( Fig. 5c ) or long time spans ( Fig. 5d ), indicating that nanostraws were responsible for the organization of these cytoskeletal elements and adhesion proteins into puncta and their colocalization. Without nanostraws, cytoskeletal behaviour was normal at long time scales [36] , as oblong paxillin structures associated with the ends of stress fibres appeared after 24 h, but the sharp paxillin puncta observed previously with nanostraws did not appear. Paxillin is but one element of focal adhesions, and additional labelling of vinculin and integrin α5 confirms frequent pair-wise colocalization of focal adhesion proteins, especially at the cell periphery ( Supplementary Fig. 9 ). Moreover, when the nanostraws were labelled with an aldehyde-fixable dye, they were found to coincide directly with GFP-paxillin ( Supplementary Fig. 10 ). The colocalization of nanostraws to paxillin and subsequent associations between paxillin and integrin, vinculin and F-actin may suggest that the nanostraws trigger downstream signalling that leads to the recruitment of adhesion proteins and F-actin complexes. While the exact role of cellular adhesion elements in nanostraw penetration requires further study to confirm, the presence of these adhesion constructs at nanostraw sites suggests that modulation of cellular adhesion can alter the nanostraw–cell interface. We have demonstrated that nanostraws can provide a fluidic pipeline into >95% of cells positioned above a microfluidic channel in order to deliver ions and small molecules directly into the cytoplasm and modulate intracellular content in real time. This direct ionic delivery was used to determine for the first time the probability with which nanowires penetrate the cell membrane, and the time scale of these processes. When coupled with the widely used toolbox of adhesion-promoting molecules, the ion delivery assay shows that improved cell adhesion greatly accelerates cell penetration while increasing the frequency of penetration. By modulating intracellular delivery by nanostraws over time, a range of natural and modified biomolecules [37] , [38] , [39] that require intracellular delivery could be applied with increased precision. For instance, the expression of a cellular protein at a particular time point can induce different behaviours than permanent genetic overexpression of the protein, which could be addressed via time-resolved nanostraw delivery [40] . This study sheds light onto previously unknown and controversial aspects of nanowire–cell interfaces. After observing the direct penetration of cells by nanostraws, we find that cellular penetration is low enough (6–12%) to make penetration difficult to observe directly, but not prohibitively low such that practical utility of the technology is limited. Each nanostraw that penetrates the cell provides sustained intracellular access, a finding that was previously unconfirmed with solid nanowire methods. Local accumulation of actin and adhesion proteins is induced around nanostraws indicating possible downstream signalling, although the exact mechanism of penetration is still unknown. These results bridge a gap between the disparate results reported by imaging studies and by functional studies, and more importantly they provide a quantitative tool to gauge progress on improving nanostraws as a biomanipulation method. Nanostraw fabrication and microfluidic assembly Nanostraws were fabricated using track-etched polycarbonate membranes with 3 × 10 7 pores cm −2 and 100-nm diameter pores (Maine Manufacturing) [16] . Membranes were coated with ~10 nm of alumina (50 cycles, atomic layer deposition, Cambridge Nanotech) and reactive ion etched in BCl 3 /Cl 2 plasma (Plasma Quest) to remove the uppermost layer of alumina, and O 2 plasma to expose the nanowires (40 min, 100 W, ~200 mTorr, Plasma Prep III Solid State, SPI Supplies). Microfluidic channels of 1 mm width and 100 μm depth were defined in polydimethylsiloxane and treated with O 2 plasma before bonding to the nanostraw device to improve device fidelity. Fabrication took place at the Stanford Nanofabrication Facility. For flow experiments, solutions were pumped at 0.1 ml min −1 (clearance time ~0.5 s) to change solutions and maintained at 0.1 ml h −1 using syringe pumps. Cell culture and imaging CHO cells were transfected with eGFP and eGFP-paxillin plasmids with Lipofectamine, selected using 200 μg ml −1 G418 and 2 μg ml −1 puromycin, respectively, and sorted using flow-assisted cell sorting (Stanford Shared FACS Facility). Cells, including CHO-B2 cells expressing α5 integrins, were maintained in Dulbecco’s modified Eagle medium supplemented with 10% fetal bovine serum, 1% penicillin/streptomycin and the aforementioned selection conditions. Before plating, cells were dissociated using 0.25% trypsin-EDTA. For confocal imaging, cells were plated on free nanostraw membranes instead of nanostraw devices, fixed in 4% paraformaldehyde and mounted using Vectashield Mounting Medium. When nanostraws were labelled with Alexa-Fluor 568 hydrazide dye, dye was added to a channel below the membrane during fixation. For vinculin staining, cells were further permeabilized with 0.25% Triton X-100 and blocked with 2% glycine, 2% bovine serum albumin, 0.2% gelatin and 50 mM NH 4 Cl in phosphate-buffered saline. Anti-vinculin mouse primary (1:1,000 dilution, 12 h incubation, 4 °C) and Alexa-Fluor 568 anti-mouse secondary (1:500 dilution, 2 h incubation, room tempareature) antibodies were used. Epifluorescence imaging of Co 2+ quenching was performed on an inverted microscope (Zeiss). Confocal imaging was performed on a spinning-disk confocal microscope (Zeiss Axiovert 200 M with a Perkin‐Elmer spinning disc and Melles Griot 43 series Ion laser), using a × 63 objective (1.4 NA, Zeiss Plan-Apochromat), photometrics Cascade 512B digital camera (Roper Scientific) and MetaMorph software (Molecular Devices). Reagents were purchased through Invitrogen. How to cite this article: Xu, A. M. et al . Quantification of nanowire penetration into living cells. Nat. Commun. 5:3613 doi: 10.1038/ncomms4613 (2014).